Polariton condensation in solitonic gap states in a one-dimensional periodic potential Manipulation of nonlinear waves in artificial periodic structures leads to spectacular spatial features, such as generation of gap solitons or onset of the Mott insulator phase transition. Cavity exciton–polaritons are strongly interacting quasiparticles offering large possibilities for potential optical technologies. Here we report their condensation in a one-dimensional microcavity with a periodic modulation. The resulting mini-band structure dramatically influences the condensation process. Contrary to non-modulated cavities, where condensates expand, here, we observe spontaneous condensation in localized gap soliton states. Depending on excitation conditions, we access different dynamical regimes: we demonstrate the formation of gap solitons either moving along the ridge or bound to the potential created by the reservoir of uncondensed excitons. We also find Josephson oscillations of gap solitons triggered between the two sides of the reservoir. This system is foreseen as a building block for polaritonic circuits, where propagation and localization are optically controlled and reconfigurable. Nonlinear wave propagation in a periodic medium is fundamentally different from the propagation in a homogeneous medium [1] . Such nonlinear waves can be photons, subject to Kerr nonlinearity ( χ 3 ), or the macroscopic wave-function of an interacting Bose–Einstein condensate. In this last case, interparticle interactions provide the equivalent of a χ 3 nonlinearity. Different localization phenomena can occur in a periodic medium due to the interplay between the band structure and interparticle interactions. In the absence of interactions, a defect state appears when the periodicity of the lattice is locally perturbed, for instance, by adding a local potential [2] , or by slightly changing the periodicity [3] or the material refractive index [4] . In the case of strong interactions or strong nonlinearities, other types of localized states, like gap solitons (GSs) [5] , [6] , [7] , [8] , [9] and truncated Bloch waves [10] , [11] , [12] , [13] can be generated, even without any perturbation of the periodic potential. GSs, typical for shallow lattice potentials, result from the interplay between the negative effective mass at the edge of the Brillouin zone and the particle repulsion. GSs possess a characteristic hyperbolic secant density profile, slowly varying in its core region and recovering an exponential decay on its edges (see Methods for details). In nonlinear photonic crystal fibres, such solitary waves have already demonstrated propagation without any distortion [14] . Besides, truncated Bloch waves have been more recently described and observed [10] , [11] , [12] , [13] . They arise in deep lattices and the localisation mechanism is self-trapping [15] , which prevents the tunnelling of particles from a strongly occupied to an empty lattice site. The spatial profile is therefore top hat-like, with exponential tails with a characteristic decay length of the order of the lattice period. Remarkably, none of these localized states can correspond to the ground state of the system. Thus, their observation with matter waves, for instance, requires setting atomic condensates out of equilibrium [7] , [8] . In the case of nonlinear photonic crystal fibres, the generation of GSs imposes to excite the system quasi-resonantly, directly inside the forbidden energy gap, which requires high excitation powers [6] . Cavity polaritons [16] are quite unique from this point of view. They are light-matter bosonic quasiparticles resulting from the strong coupling between photons and excitons in semiconductor structures [16] . Polariton condensation has been demonstrated [17] , [18] , [19] , [20] , [21] , [22] together with many nonlinear phenomena, such as formation of quantized vortices [23] and solitons [24] , [25] or superfluidity [26] . The optical nonlinearities associated with polariton–polariton interactions are typically orders of magnitude larger than in other nonlinear optical systems [27] . Moreover, modern lithography techniques open large possibilities in potential engineering [28] , [29] , [30] . Owing to their finite lifetime, polaritons can demonstrate out-of-equilibrium features and the quantum state in which condensation occurs is not necessarily the ground state [30] . It strongly depends on the relative efficiency of relaxation from the excitonic reservoir towards the different accessible states [30] . In particular, condensation phenomena in one dimensional (1D) wires, driven by a tightly focused laser spot, have been shown to generate finite momentum condensates, ballistically expanding from the injection area along the wire [31] . This expansion was driven by the repulsive potential induced by the excitonic reservoir localized in the pump region. In the present work, we show that in a 1D periodic potential under similar excitation conditions, polaritons spontaneously condense into highly localized GS states. Depending on the experimental configuration, these GSs can be either bound to the potential created by the pump-induced excitonic reservoir, or free to propagate away from the excitation area. GSs bound to each side of the reservoir can hybridize into a symmetric (bonding state S2) and anti-symmetric (anti-bonding state S1) linear combinations. Condensation in either of these two states S1 or S2 can be favored controlling the excitation conditions. Under pulsed excitation, we could achieve excitation of a linear combination of S1 and S2, resulting in spatial oscillations of the GS from one side of the reservoir to the other. This behavior can be understood as Josephson oscillations of GSs across the tunnel barrier defined by the excitonic reservoir. At large pumping powers, efficient depletion of the reservoir into the condensate allows unbinding and propagation of the GSs. All these experiments are well described by a model including the coupled dynamics of both the reservoir and the polariton condensate [30] . These results highlight the potentiality of this strongly nonlinear photonic system to generate and manipulate GSs. Structure and band profile We have designed an original cavity microstructure to generate polaritons in a quasi 1D periodic potential. We benefit from the mixed nature of the polariton states, creating a periodic potential by engineering of the photonic component, and making use of the interactions brought by the excitonic part. Starting from a planar cavity with high quality factor (polariton lifetime exceeding 40 ps), we fabricated wires with a periodically modulated width (see Fig. 1a ), thus inducing a periodic modulation of amplitude V opt of the cavity mode energy. This creates a periodic potential for the polariton state, with an amplitude proportional to the modulation width. The ratio between the recoil energy ( m is the polariton mass and P is the lattice period) and V opt is of the order of 1 or slightly smaller in our samples, which favors the formation of GSs rather than of truncated Bloch waves. As evidenced by far-field emission measurements and calculation in the low-density regime (see Fig. 1b–d ), this periodic potential results in the formation of polariton mini-bands separated by mini-gaps. The edge of the 1st Brillouin zone is at π / P and the width of the mini-gaps is determined by the amplitude of the modulation. We note that, differently from previously reported techniques used to spatially modulate the polariton energy [32] , [33] , [34] , the resulting amplitude of the potential is much larger and can potentially be as large as several millielectronvolts. 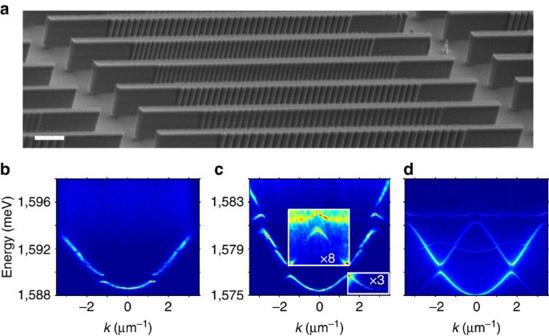Figure 1: Polariton dispersion in modulated microwires. (a) Scanning electron microscopy image of an array of laterally modulated wires; the white scale bar corresponds to a length of 10 μm. (b) Angle-resolved emission measured on a single modulated wire in the low density regime; the modulation period isP=2.7 μm and the wire width is modulated betweenWmin=1.9 μm andWmax=2.8 μm, inducing a periodic potential of amplitudeVopt=1.6 meV on the cavity mode, the detuning isδ=−1 meV (Ec=1,595.5 meV,Ex=1,596.5 meV). (c) Same as (b) withP=2.1 μm,Wmin=1.8 μm andWmax=3.5 μm inducing a periodic potentialVopt=2.4 meV,δ=−9.5 meV (Ec=1,579.5 meV,Ex=1,589 meV). The signal inside the rectangles has been amplified to better show the band folding. (d) Simulated polariton dispersion of the wire shown in (c). Figure 1: Polariton dispersion in modulated microwires. ( a ) Scanning electron microscopy image of an array of laterally modulated wires; the white scale bar corresponds to a length of 10 μm. ( b ) Angle-resolved emission measured on a single modulated wire in the low density regime; the modulation period is P =2.7 μm and the wire width is modulated between W min =1.9 μm and W max =2.8 μm, inducing a periodic potential of amplitude V opt =1.6 meV on the cavity mode, the detuning is δ =−1 meV ( E c =1,595.5 meV, E x =1,596.5 meV). ( c ) Same as ( b ) with P =2.1 μm, W min =1.8 μm and W max =3.5 μm inducing a periodic potential V opt =2.4 meV, δ =−9.5 meV ( E c =1,579.5 meV, E x =1,589 meV). The signal inside the rectangles has been amplified to better show the band folding. ( d ) Simulated polariton dispersion of the wire shown in ( c ). Full size image Theoretical background on GSs bound to a potential barrier In the experiments we report, polaritons are generated under non-resonant optical excitation, either continuous wave (cw) or pulsed, by a laser focused down to a 2-μm diameter spot. Such injection conditions locally create a high density of excitons, named the excitonic reservoir, forming a local repulsive potential for the polaritons. Depending on the relative strength of this potential as compared with the interaction energy, the nature of the gap states in the periodic medium is strongly affected: far from the local potential, free GSs can exist and are described by the standard GS wave function. They present a hyperbolic secant profile with a characteristic size, which decreases when going from the low density (bottom of the gap) to the high density limit (centre of the gap). To illustrate the effect of the local excitonic potential, bound GS states can be found analytically, considering a simple delta potential V 0 δ ( x ) for the reservoir (see Methods for details and analytical expression of the envelope function of the GSs). Changing the ratio ( α being the interaction constant and N the number of particles within the soliton) while keeping the energy E =| m |( V 0 + αN /2) 2 /2 ħ 2 constant, one obtains a family of degenerate bound states with different spatial profiles. In the absence of interactions ( N =0), the wave function of the localized state decays exponentially in space. By increasing the density, the state broadens, changes its shape and the wave function approaches the one of a free GS. The left part of Fig. 2a shows the envelope of such wave functions for an energy close to the lower edge of the gap and for three particle densities. It illustrates this progressive change in the GS spatial shape. Let us underline that even weak nonlinearities, corresponding to energy shifts of a few tens of microelectronvolts, produce significant changes in the density profile. The right part of the image corresponds to a larger energy, and results in shorter localization length. In this case, the shape of the GSs is not significantly affected by the ratio . 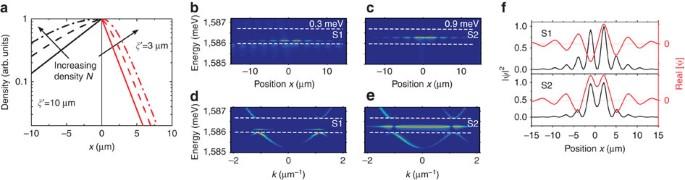Figure 2: Gap soliton states bound to a delta potential. (a) Envelope of GS wave functions bound to a defect, calculated using formula (2) to (5) with different parameters. Left side:ξ'=10 μm,E=10 μeV. Solid line:αN=0, dashed lineαN=12 μeV·μm, dotted dashedαN≈20 μeV·μm. Right sideξ'=3 μm,E=100 μeV, solid line:αN=0, dashed lineαN≈120 μeV·μm, dotted dashedαN≈200 μeV·μm. (b,c) and (d,e) Calculated emission distribution in real and ink-space solving the time-dependent Schrödinger equation including pumping and lifetime, in the presence of both a periodic potential and a Gaussian potential atx=0 μm and of height (b,d) 0.3 meV, and (c,e) 0.9 meV. The pumping is a delta function in time and space which allows exciting the more localized solutions of the spectrum. The white dashed lines indicates the position of the first energy mini-gap induced by the period potential. (f) Density probability (black line) and real part of the S1 (up) and S2 (down) wavefunctions, showing respectively the anti-symmetric and symmetric character with respect to the reservoir position. (The imaginary parts present the same symmetries.) Figure 2: Gap soliton states bound to a delta potential. ( a ) Envelope of GS wave functions bound to a defect, calculated using formula (2) to (5) with different parameters. Left side: ξ' =10 μm, E =10 μeV. Solid line: αN =0, dashed line αN =12 μeV·μm, dotted dashed αN ≈20 μeV·μm. Right side ξ' =3 μm, E =100 μeV, solid line: αN =0, dashed line αN ≈120 μeV·μm, dotted dashed αN ≈200 μeV·μm. ( b , c ) and ( d , e ) Calculated emission distribution in real and in k -space solving the time-dependent Schrödinger equation including pumping and lifetime, in the presence of both a periodic potential and a Gaussian potential at x =0 μm and of height ( b , d ) 0.3 meV, and ( c , e ) 0.9 meV. The pumping is a delta function in time and space which allows exciting the more localized solutions of the spectrum. The white dashed lines indicates the position of the first energy mini-gap induced by the period potential. ( f ) Density probability (black line) and real part of the S1 (up) and S2 (down) wavefunctions, showing respectively the anti-symmetric and symmetric character with respect to the reservoir position. (The imaginary parts present the same symmetries.) Full size image We have also computed the GS profile, considering a more realistic Gaussian barrier instead of a delta potential. We found that the GSs solutions arise from the coupling of localized states on each side of the potential: this coupling leads to the formation of an anti-symmetric anti-bonding state S1 and a symmetric bonding state S2. The panels of Fig. 2b (respectively d,e) show examples of calculated eigenfunctions in real (respectively reciprocal) space in the case of weak interaction regime ( αN << V 0 ). For a weak potential ( Fig. 2b ), the anti-bonding state S1 is observed in the gap, while for larger potential value ( Fig. 2c ), the symmetric bonding-state S2 dominates. The symmetric and anti-symmetric character of the wavefunctions is illustrated in Fig. 2f . When interactions are increased in the model, the envelope spatial shape of these localized states varies with the ratio in the same way as discussed above. Condensation in bound GS states under cw excitation Let us address cw excitation conditions where polaritons are excited non-resonantly using a single-mode cw laser tuned typically 100 meV above the bottom of the polariton lower branch. We consider the case where the laser spot is centred onto a barrier region of the periodic potential (as shown in the inset of Fig. 3b ). Increasing the excitation power, we observe a sharp threshold in the emission intensity, signature of polariton condensation (see Fig. 3a ). Below threshold power ( P th ), the real space distribution of the polariton emission shows delocalized states, and demonstrates propagation of polaritons in the different sub-bands ( Fig. 3b ). Above threshold, real and reciprocal space images show that the condensation takes place in a gap state S1, just above threshold ( Fig. 3c ), and in the gap state S2 for higher pumping power ( Fig. 3d ). Condensation is triggered on these excited states rather than on lower energy states of the first allowed band, because these localized states have the largest spatial overlap with the excitonic reservoir, providing efficient relaxation kinetics. When we excite on a barrier, the S1 gap state is found at a higher energy than the symmetric S2 state. Close to threshold, the S1 energy lies close to the centre of the gap, whereas S2 is closer to the lower band edge. The state S1 is therefore much more localized, and as result, better coupled to the reservoir. Condensation is triggered on S1 because it is kinetically favored. For higher pumping rates, both S1 and S2 blueshift. S2 becomes more localized than S1, and is eventually favored. These experiments show that counter-intuitively, repulsive interactions lead to the condensate localization in presence of a periodic potential. While it is known that disorder can also strongly affect the propagation of polariton condensates [31] provoking localization phenomena [35] , the data taken below the condensation threshold ( Fig. 3b ) demonstrate the propagation of polaritons over tens of microns. The localization arising in the condensation regime happens on a much shorter scale (2–7 μm) and is not likely to be induced or even strongly affected by disorder. The spatial emission profile of the two modes S1 and S2 is shown on the Fig. 3h . The state S2, energetically close to the centre of the gap, shows a short localization around 2 μm, close to P =2.7 μm. One should note that for such energy in the gap, this is the typical size expected both for a state localized by the presence of the reservoir and for a pure GS state. Therefore it is difficult to distinguish between the two localization mechanisms. The situation is different for state S1, being located at lower energy, and thus being wider (around 6 μm). S1 shows the characteristic hyperbolic secant profile, signature of the role of polariton interactions in the localization feature. Finally, let us mention that condensation in the gap state S2 can also be triggered by moving the excitation spot into a local minimum of the periodic potential (this effect will be illustrated for pulsed excitation in the following). 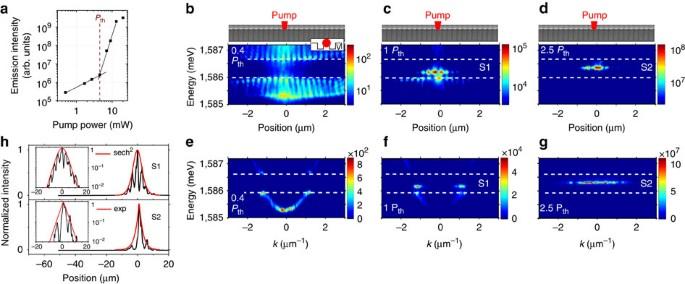Figure 3: Condensation in solitonic gap states under cw excitation. A modulated wire is excited with a 2-μm cw laser spot centered on a maximum of the periodic potential (narrow region of the wire). (a) Total emission intensity measured from a single modulated wire as a function of the excitation power. (b–d) Spectrally and spatially resolved emission for three excitation powers (in logarithmic color scale). The inset of (b) illustrates the position of the pumping spot centered onto a maximum of the periodic potential. (e–g) Spectrally resolved far-field emission measured on the same wire for the same excitation powers (in linear color scale); the first mini-gap induced by the periodicity is indicated with dashed lines. The intensity profile of the states S1 and S2 is shown in panel (h). The measured FWHM of S1 and S2 are 6.1 μm and 2.2 μm. S1 is fitted by a sech2envelope function (eq. (1) in the text), S2 with an exponential. In the insets, the same profiles are shown in log scale. (Parameters of the wire: period 2.7 μm,Wmin=1.9 μm andWmax=2.8 μmVopt=1.6 meV;δ=−5.5 meV (Ec=1,590.5 meV,Ex=1,596 meV)). Figure 3: Condensation in solitonic gap states under cw excitation. A modulated wire is excited with a 2-μm cw laser spot centered on a maximum of the periodic potential (narrow region of the wire). ( a ) Total emission intensity measured from a single modulated wire as a function of the excitation power. ( b – d ) Spectrally and spatially resolved emission for three excitation powers (in logarithmic color scale). The inset of ( b ) illustrates the position of the pumping spot centered onto a maximum of the periodic potential. ( e – g ) Spectrally resolved far-field emission measured on the same wire for the same excitation powers (in linear color scale); the first mini-gap induced by the periodicity is indicated with dashed lines. The intensity profile of the states S1 and S2 is shown in panel ( h ). The measured FWHM of S1 and S2 are 6.1 μm and 2.2 μm. S1 is fitted by a sech 2 envelope function (eq. (1) in the text), S2 with an exponential. In the insets, the same profiles are shown in log scale. (Parameters of the wire: period 2.7 μm, W min =1.9 μm and W max =2.8 μm V opt =1.6 meV; δ =−5.5 meV ( E c =1,590.5 meV, E x =1,596 meV)). Full size image Dynamics of GSs under pulsed excitation In the rest of the paper, we consider pulsed excitation conditions and monitor the emission with a picosecond time resolution. This allows revealing the formation and the dynamics of GSs. In this experimental scheme, the exciton reservoir is populated by a picosecond pulse. While the free decay time of the exciton reservoir is of the order of 400 ps, it can be much faster in the condensation regime, when a rapid transfer of particles into the condensed state occurs. Depending on the excitation conditions (pump power and location of the excitation beam), we obtained interesting and qualitatively distinct dynamical regimes, which are described below. 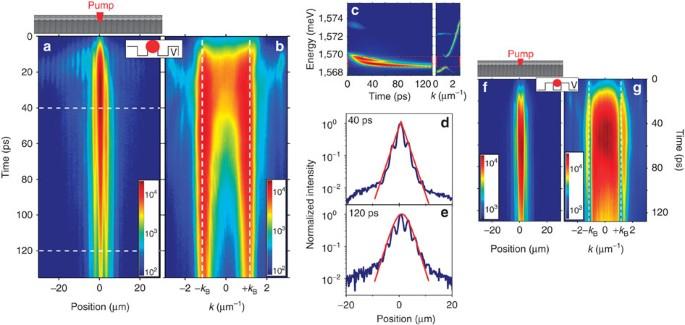Figure 4: Dynamical condensation in solitonic gap states. A modulated wire is excited with a 2-μm pulsed laser spot centered on a maximum of the periodic potential withP=2.5Pth. (a) Spatially resolved emission measured as a function of time. (b) Reciprocal space emission as a function of time. The dashed lines show the position of the edges of the first Brillouin zone. (c) Energy of the emission as a function of time measured at the center of the wire. The horizontal red dashed lines shows the position of the first gap, which is extracted from the energy resolved measurements at low excitation density shown on the right part of the panel. (d,e) Normalized spatial profile of the emission extracted from (a) at different times (corresponding to the white dashed lines in (a)), in red line are shown fits of the central part (d) by an exponential and (e) a sech2envelope function (withξ=3.3 μm (see eq. (1))). (f,g) Same as (a) and (b) but with the laser spot centered on a minimum of the periodic potential. (Parameters of the considered wire: period 2.7 μm,Wmin=1.9 μm andWmax=2.8 μmVopt=1.6 meV;δ=−7.5 meV (Ec=1,573 meV,Ex=1,580.5 meV).) Figure 4a–e shows data taken at 2.5 P th , with the laser positioned on a potential barrier. Here, we evidence the formation of a quasi-stationary GS in the state S1. For short time delays, a small part of the emission lies in the second allowed band ( Fig. 4c ) and the corresponding real space image indeed shows a weak signal propagating away from the excitation spot, reminiscent of the condensate expansion in flat wires [28] . Figure 4: Dynamical condensation in solitonic gap states. A modulated wire is excited with a 2-μm pulsed laser spot centered on a maximum of the periodic potential with P =2.5 P th . ( a ) Spatially resolved emission measured as a function of time. ( b ) Reciprocal space emission as a function of time. The dashed lines show the position of the edges of the first Brillouin zone. ( c ) Energy of the emission as a function of time measured at the center of the wire. The horizontal red dashed lines shows the position of the first gap, which is extracted from the energy resolved measurements at low excitation density shown on the right part of the panel. ( d , e ) Normalized spatial profile of the emission extracted from ( a ) at different times (corresponding to the white dashed lines in ( a )), in red line are shown fits of the central part ( d ) by an exponential and ( e ) a sech 2 envelope function (with ξ= 3.3 μm (see eq. (1))). ( f , g ) Same as ( a ) and ( b ) but with the laser spot centered on a minimum of the periodic potential. (Parameters of the considered wire: period 2.7 μm, W min =1.9 μm and W max =2.8 μm V opt =1.6 meV; δ =−7.5 meV ( E c =1,573 meV, E x =1,580.5 meV).) Full size image After 20 ps, most of the emission arises at an energy inside the gap (see Fig. 4c ), slowly decreasing and reaching the bottom of the gap at a longer time. The reciprocal space emission is composed of two harmonics located at the edges of the Brillouin zone ± k B ( Fig. 4b ), which is a characteristic of the S1 GS (see Fig. 2d ). The corresponding spatial emission is strongly localized at short times and the profiles can be well fitted by an exponential up to 40 ps ( Fig. 4d ), indicating that localisation is driven by the reservoir. At longer time, the shape of the emission changes and is well fitted with a hyperbolic secant envelope function ( Fig. 4e ): this is the signature of the role of polariton self-interactions in the formation of the GS. The GS remains immobile, fed by the exciton reservoir and bound to its potential. Spontaneous formation of a GS in the S2 state, with similar dynamics than in the case just described, can be obtained for the same excitation power, when centring the excitation spot onto a minimum of the periodic potential ( Fig. 4f ). The characteristic far-field pattern of S2 with two minima at ± k B is then observed ( Fig. 4g ). Interestingly, a more complex dynamical regime can be obtained when placing the laser spot at the edge of a potential barrier. Under such excitation conditions, condensation is triggered towards a linear combination of the states S1 and S2. We then observe pronounced oscillations both in real and reciprocal space ( Fig. 5a ), while the emission energy always remains within the gap ( Fig. 5c ). The GS moves from one side of the reservoir to the other one, passing through the tunnel barrier induced by the excitonic reservoir. This effect is similar to Bosonic Josephson oscillations [36] , [37] , [38] , observed here for the first time with GSs. Let us mention that the spatial amplitude of the oscillations can be increased by using larger pumping powers or pump spot (not shown). 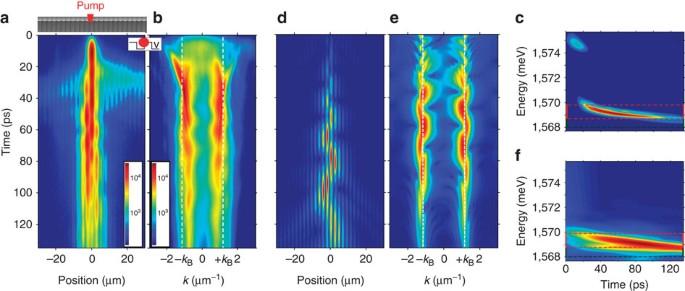Figure 5: Josephson oscillations of gap solitons. A modulated wire is excited with a 2 μm pulsed laser spot positioned in between a minimum and a maximum of the periodic potential.P=4Pth(a,b) Spatial and reciprocal space emission as a function of time. (c) Energy of the emission as a function of time measured at the center of the wire. (d,e) Simulation of the time evolution of the emission (d) in real space and (e) in reciprocal space, obtained using the model described in the Methods section. (f) Calculated emission energy as a function of time obtained in this simulation. Figure 5d–f presents the results of a simulation reproducing these excitation conditions. We use a model of polariton condensation, similar to the one presented in the study of Wertz et al . [39] We consider the coupling between a local exciton reservoir and the condensate, whose evolution is described by the Gross–Pitaevskii equation (see Methods for details). Good overall agreement with the experimental observation is obtained despite the configuration complexity. Figure 5: Josephson oscillations of gap solitons. A modulated wire is excited with a 2 μm pulsed laser spot positioned in between a minimum and a maximum of the periodic potential. P =4 P th ( a , b ) Spatial and reciprocal space emission as a function of time. ( c ) Energy of the emission as a function of time measured at the center of the wire. ( d , e ) Simulation of the time evolution of the emission ( d ) in real space and ( e ) in reciprocal space, obtained using the model described in the Methods section. ( f ) Calculated emission energy as a function of time obtained in this simulation. Full size image Finally we want to consider higher excitation conditions where the excitonic reservoir can be strongly depleted because of fast transfer of particles into the polaritonic GS. 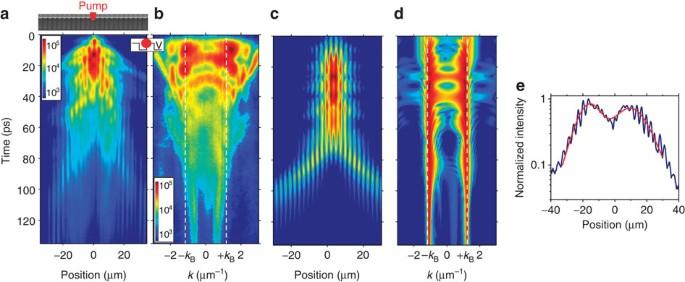Figure 6: Dynamical unbinding of gap solitons. A modulated wire is excited with a 2 μm pulsed laser spot positioned in between a minimum and a maximum of the periodic potential.P=10Pth. (a,b) Spatial and reciprocal space emission as a function of time. (c,d) Simulation of the time evolution of the emission (c) in real space and (d) in reciprocal space, obtained in these high excitation conditions using the model described in the Methods section; (e) Normalized real space profile of the emission extracted from (a) at a time delay of 80 ps (blue line); the red line corresponds to a fit with the sum of two sech2envelope functions withξ=10 μm (see eq. (1)). (Wire parameters same asFigs 4and5, withδ=−3 meV (Ec=1,587 meV,Ex=1,590 meV).) Figure 6 presents measurements obtained with excitation conditions similar to that of Fig. 5 , but for a higher pumping power (10 P th ). At short times, a complex behavior both in real and k -space is observed, due to ballistic propagation of high energy polaritons, together with GS oscillations similar to the case described in Fig. 5 . Interestingly, after 50–60 ps, the signal in the excitation area vanishes. This is the signature of significant depletion of the excitonic reservoir due to stimulated transfer into the GS. Thus, the reservoir potential is strongly reduced: GS unbinds on each side of the excitation area and starts to propagate away (see Fig. 6a ). This unbinding is accompanied by a broadening of the GS: its polariton density decreases as it is no more populated by the reservoir. Figures 6c present simulations corresponding to this high-density regime using our model. Contrary to the experiments, the simulation does not populate states in the second allowed energy band and so the propagating behavior and high k -values emission observed before 40 ps can of course not be reproduced by our model. Nevertheless unbinding and propagation of gap solitons at longer time delays is predicted in qualitative agreement with the experiment. This regime could be of high importance for future applications. It shows that a bound GS can be created via non-resonant excitation, and then released as a free nonlinear wave pulse, useful for information transfer. Figure 6: Dynamical unbinding of gap solitons. A modulated wire is excited with a 2 μm pulsed laser spot positioned in between a minimum and a maximum of the periodic potential. P =10 P th . ( a , b ) Spatial and reciprocal space emission as a function of time. ( c , d ) Simulation of the time evolution of the emission ( c ) in real space and ( d ) in reciprocal space, obtained in these high excitation conditions using the model described in the Methods section; ( e ) Normalized real space profile of the emission extracted from ( a ) at a time delay of 80 ps (blue line); the red line corresponds to a fit with the sum of two sech 2 envelope functions with ξ= 10 μm (see eq. (1)). (Wire parameters same as Figs 4 and 5 , with δ =−3 meV ( E c =1,587 meV, E x =1,590 meV).) Full size image Our time-resolved experiments under non-resonant excitation provide a very effective and simple way to create polariton condensates in the form of gap solitons and to study and control their dynamics. This is in contrast with standard photonic systems, where the excitation of GSs requires complex strategies using resonant beams. The polaritonic GSs could be further manipulated, for instance, by using several control beams in fully reconfigurable polaritonic circuits. In such a way, the information could be stored in polaritonic GSs, then released, and eventually transmitted in an ultrafast way. Interestingly, the photonic potential engineered in the present work, imposes periodic modulation of the exciton fraction of the polariton and, therefore, of the effective interaction constant. Our system thus represents a practical implementation of mixed linear/nonlinear lattices, where an extremely rich phenomenology has been found theoretically in the recent years [40] . Sample and measurements The sample consists in a λ /2 Ga 0.05 Al 0.95 As cavity embedded between two Ga 0.05 Al 0.95 As/Ga 0.8 Al 0.2 As Bragg mirrors with respectively 40 (28) pairs in the bottom (top) mirror. The nominal quality factor is around 10 5 . Three sets of four 7-nm GaAs quantum wells are inserted at the antinodes of the electromagnetic field resulting in a 15-meV Rabi splitting. 120 microns-long modulated wires were fabricated using electron-beam lithography and dry etching. We define the exciton–photon detuning as δ = E c – E x , where E c and E x are the cavity mode and exciton energy at k || =0, respectively. Measurements have been performed on several wires at different regions of the sample. The presence of a gradient of both the quantum well width and of the cavity width gives access to a wide range of detuning δ and, at the same time, to iso-detuned polaritons at different energies. This explains the small difference in absolute energy from one figure to the other. Micro-photoluminescence measurements are performed at 10 K. For the cw measurements, the excitation is provided by a single-mode Ti:sapphire laser. The emission is detected by a nitrogen-cooled CCD camera. For the pulsed experiments, a Ti:sapphire laser delivering 1.4-ps pulses with a 80-MHz repetition rate is used. Time-resolved emission is monitored using a synchroscan streak camera, with an overall time resolution of 6 ps. The far (respectively near)-field spectroscopy is obtained projecting the Fourier plane of the detection microscope objective (respectively, the sample surface plane) on the entrance slit of a monochromator, placed prior to the CCD camera or to the streak camera. Theory of gap solitons bound to a defect potential GSs arise from the interference between two counter propagating wave packets having their central wave vectors at the edges of the Brillouin zone, ± k B =± π / P . The corresponding wave function reads in real and reciprocal space: Here, is the healing length, where α is the polariton–polariton interaction constant [41] , [42] , m is the polariton mass, n 0 =| ψ (0) 2 | the soliton peak density in real space. In reciprocal space, a GS wave function therefore exhibits two symmetric maxima at ± k B , which contrasts with the wave function of truncated Bloch waves that always exhibits a maximum at k =0. GSs are stationary solutions of the Gross–Pitaevskii equation for energies lying between the bottom and the middle of the first gap. Their healing length decreases from infinity at the band edge (low density) up to the lattice period at the centre of the gap (for higher densities). GSs bound to a defect We consider particles of negative mass m , given by the curvature of the dispersion at the edge of the Brillouin zone. The interaction constant is repulsive. A simple analytical solution of the Gross–Pitaevskii equation in the presence of a spatial potential V 0 δ ( x ) is given by a truncated GS wave function: This solution is obtained from matching conditions: the jump of the derivative at the barrier is proportional to the strength of the barrier potential, and in other points, the free GS solution remains unperturbed. The characteristic decay length of the wave envelope function is linked to the energy of the state as: where the energy above the edge of the conduction band is given by and N is the total number of particles in the GS. The truncation coordinate x 0 can be found as: In the non-interacting case, x 0 →∞, and the wave function is an exponentially decaying defect state. In the case of strong interactions, α N /2 V 0 →∞, x 0 →0, and we recover a free GS wave function. A continuous transformation from an exponential defect state to a free GS is obtained when increasing and keeping the quantity constant, and thus, the energy. This effect is illustrated in Fig. 2a . Model of polariton relaxation In order to simulate the experiment performed under non-resonant pumping, we used the Gross–Pitaevskii equation for the condensate with relaxation terms accounting for polariton–polariton scattering, coupled with the equation for the reservoir, similar to the study of Wertz et al . [39] , where the same model was applied to unmodulated wires. Here ψ ( x , t ) is the condensate wavefunction, n R ( x , t ) is the reservoir density, m =4.5 × 10 −5 m 0 is the polariton mass ( m 0 is the free-electron mass), τ pol =40 ps is the polariton lifetime. is the polariton–polariton interaction constant, where E b =6 meV is the exciton binding energy; =10 nm, the exciton Bohr radius and W =2.3 μm, the average wire width. D =5 × 10 −2 μm 2 ps −1 is the exciton diffusion coefficient, τ R =400 ps is the reservoir lifetime, P ( t ) is the pulsed non-resonant pumping (particles are injected at t =0), and σ =1 μm is the width of the pumping spot. γ =3 × 10 9 μm s −1 describes stimulated scattering from the reservoir to the condensate; the last term of equation (6) with a fitting parameter Λ 0 =10 −3 describes the energy relaxation of the polariton condensate induced by interactions with the thermalized excitonic reservoir. D.T., A.A. and J.B. performed the experiments and analyzed the data. H.F., D.S. and G.M. carried out the theoretical analysis and simulations. A.L., E.G., R.B., P.S. and I.S. worked on the growth and etching of the sample. All of the authors designed the experiment, discussed the underlying physics and contributed to the manuscript. How to cite this article: Tanese, D. et al . polariton condensation in solitonic gap states in a one-dimensional periodic potential . Nat. Commun. 4:1749 doi: 10.1038/ncomms2760 (2013).